Site-specific Umpolung amidation of carboxylic acids via triplet synergistic catalysis Development of catalytic amide bond-forming methods is important because they could potentially address the existing limitations of classical methods using superstoichiometric activating reagents. In this paper, we disclose an Umpolung amidation reaction of carboxylic acids with nitroarenes and nitroalkanes enabled by the triplet synergistic catalysis of FeI 2 , P(V)/P(III) and photoredox catalysis, which avoids the production of byproducts from stoichiometric coupling reagents. A wide range of carboxylic acids, including aliphatic, aromatic and alkenyl acids participate smoothly in such reactions, generating structurally diverse amides in good yields (86 examples, up to 97% yield). This Umpolung amidation strategy opens a method to address challenging regioselectivity issues between nucleophilic functional groups, and complements the functional group compatibility of the classical amidation protocols. The synthetic robustness of the reaction is demonstrated by late-stage modification of complex molecules and gram-scale applications. The amide functional group is an important moiety present in a broad spectrum of biologically active compounds, synthetic materials and building blocks [1] , [2] . About 25% of natural and synthetic drugs on the market contain at least one amide [3] and consequently, the development of new synthetic strategy for the construction of amide bonds is pivotal in both organic synthesis and pharmaceutical production [4] , [5] , [6] . In addition to the biosynthetic routes [7] , classical synthetic routes from readily available carboxylic acids generally require either reagents which can activate carboxylic acids or preparation of reactive intermediates, such as esters, anhydrides or acyl chlorides for subsequent amidation with nucleophilic amines (Fig. 1a ) [8] , [9] , [10] , [11] , [12] , [13] , [14] , [15] , [16] , [17] , [18] , [19] . Nitroarenes are readily available and cheap feedstock reagents [20] , [21] , [22] , [23] , [24] , [25] , [26] , [27] and have recently been applied with reduction in situ as amination reagents in amidation [28] , [29] , [30] . For example, Ma et al. recently achieved an elegant one-pot stoichiometric amidation protocol of carboxylic acids with nitroarenes [30] . Although these typical amide bond formation strategies are powerful, the development of a catalytic amidation protocol of carboxylic acids is still being actively pursued in the context of sustainable synthetic chemistry [1] , [31] as the carboxylic acid activating reagents not only result in some harmful byproducts but also would compromise the functional group tolerance. Fig. 1: The state-of-the-art of amidation of carboxylic acids. a Well-established amidation protocols of carboxylic acids. b Iron/P(III)/Photoredox catalysis for Umpolung amidation. PC photocatalyst. Full size image Recently, our group developed a photoredox, Ph 3 P radical cation-mediated deoxygenation of aromatic acids, generating the corresponding acyl radical which participates in a series of novel organic transformations [32] , [33] , [34] . At the same time, Doyle and others also disclosed a similar activation mode of carboxylic acids [35] , [36] , [37] . However the use of stoichiometric amounts of Ph 3 P will diminish the total reaction economy, leading to issues in purification, and the aliphatic carboxylic acids remain challenging substrates with Ph 3 P as deoxygenation reagent under photoredox conditions due to the possibility of their decarboxylation [38] , [39] , [40] , [41] . Inspired by Radosevich’s recent seminal work on the P(III)/P(V) catalytic cycle [25] , [42] , [43] , [44] , [45] , [46] , we questioned if Umpolung amidation of carboxylic acids is possible with electrophilic amination reagents of nitroarenes. Such a reaction could proceed by means of synergistic photoredox and R 3 P/R 3 P = O catalysis, where the generated nucleophilic acyl radical undergoes radical addition to electrophilic amination reagents as shown in Fig. 1b . This kind of amide bond formation strategy would avoid the use of nucleophilic amine reagents and address the regioselectivity issue between different amine motifs, thus improving the functional group compatibility. A significant difficulty for the Umpolung amidation originates from the fact that the reaction rates between carboxylic C-O homolysis, R 3 P = O and nitroarenes reduction should be matched to support the concerted catalytic cycles. Herein we report an Umpolung amidation strategy of various carboxylic acids with commercially abundant nitroarenes and nitroalkanes by means of iron/R 3 P/photoredox multi-cooperative catalysis. Reaction optimization Initially, we selected n -heptanoic acid ( 1a ) and nitrobenzene ( 2a ) as model reactants with which to investigate the Umpolung amidation conditions. 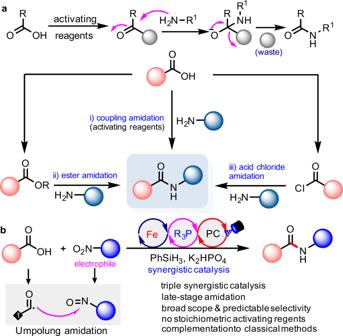Fig. 1: The state-of-the-art of amidation of carboxylic acids. aWell-established amidation protocols of carboxylic acids.bIron/P(III)/Photoredox catalysis for Umpolung amidation. PC photocatalyst. As shown in Table 1 , the standard conditions include synergistic catalysis by 15 mol% FeI 2 , 30 mol% organophosphine ( P-A ) and 1 mol% PC-I in the presence of PhSiH 3 as the reductant (entry 1, also see Supplementary Information for details). 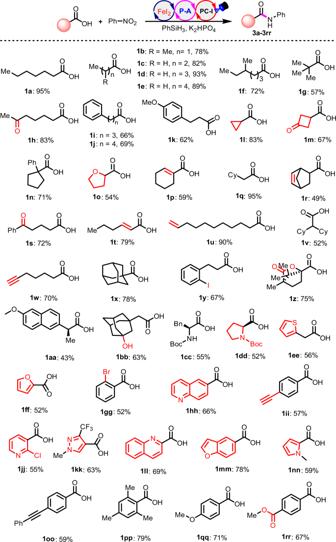Fig. 2: The scope of carboxylic acids. Standard conditions: carboxylic acids1(0.2 mmol),2a(1.2 equiv),PC-I(1 mol%),P-A(30 mol%), FeI2(15 mol%), K2HPO4(0.5 equiv), PhSiH3(1 mmol), MeCN (4 ml), blue LEDs, ambient temperature, 24-40 h. Under the standard conditions, the desired amide ( 3a ) is obtained in 95% isolated yield. The use of other organophosphine precatalysts ranging from P-B to P-F significantly decreased the reaction efficiency (entries 2-6). We presumed that P-A (R 3 P = O) undergoes rapid reduction rates in the presence of FeI 2 and silanes to generate R 3 P at room temperature [47] , [48] , [49] . Replacement of FeI 2 with other iron-based catalysts also led to sharply decreased yields (entries 7 and 8). It was speculated that iron-based catalysts would not only accelerate the reduction of R 3 P = O to R 3 P but would also favor the reduction of nitrobenzene to nitrosobenzene under mild conditions [26] , [50] , [51] , [52] . 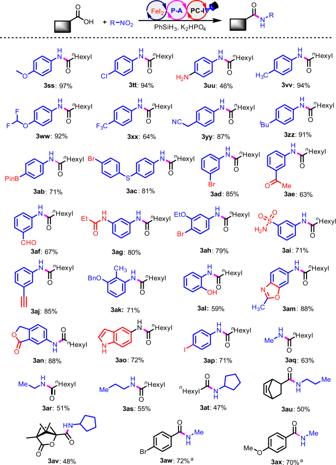Fig. 3: The scope of the organonitro compounds. Standard conditions:1a(0.2 mmol), R-NO22(0.24 mmol),PC-I(1 mol%),P-A(30 mol%), FeI2(15 mol%), K2HPO4(0.5 equiv), PhSiH3(1 mmol), MeCN (4 ml), blue LEDs, ambient temperature, 24-36 h.a2.0 equivalent nitromethane was used. Notably, the use of other silanes in place of PhSiH 3 did not improve the reaction yields (entries 9 and 10, and also see Supplementary Table 3 for details). Control experiments suggested that all the factors, FeI 2 , organophosphine precatalyst, photocatalyst and light irradiation were important for the successful Umpolung amidation (entries 11-14). The triplet catalytic systems should work in concert to meet the total reaction rate demand. A single faster or slower catalytic cycle will mismatch the synergistic effect, thus negatively influencing the reaction. Table 1 Optimization of catalytic Umpolung amidation conditions a . Full size table Substrate scope With the optimal conditions in hand, we explored the substrate scope of carboxylic acids. As can be seen in Fig. 2 , this Umpolung amidation has a satisfactory functional group compatibility and a broad carboxylic acid substrate scope. A series of structurally diverse carboxylic acids ( 1a-1rr ) are competent starting materials, affording the desired amides ( 3a-3rr ) in moderate to good yields (44 examples, up to 95% yield). Primary, secondary and tertiary aliphatic acids ( 1a-1o , 1q-1s , 1u-1ee ) all tolerate the conditions well and the protocol has excellent functional group tolerance. A great number of versatile functional groups, such as ketone ( 1 h , 1 m, 1 s ), iodo ( 1 y ), bromo ( 1gg ), cyclopropanyl ( 1 l ), alkene ( 1p , 1r , 1 u ), alkyne ( 1w, 1ii ), ester ( 1z ), heterocycle ( 1o , 1dd - 1ff , 1hh, 1jj-1nn ) remain intact. Besides aliphatic carboxylic acids, α,β-unsaturated acids ( 1p and 1t ) and aromatic acids ( 1gg-1ii, 1oo-1rr ) as well as heteroaromatic acids ( 1ff , 1jj-1nn ) are also efficient coupling partners and can be directly employed for the construction of the corresponding amides. Interestingly, when the chiral amino acids ( 1cc and 1dd ) were subjected to this protocol, the chiral amides were obtained without racemization as determined by HPLC analysis. The use of organophosphine precatalyst ( P-A) as the deoxygenation catalyst appears to complement Ph 3 P-mediated deoxygenative coupling, significantly expanding the carboxylic acid scope [32] , [33] , [34] . Fig. 2: The scope of carboxylic acids. Standard conditions: carboxylic acids 1 (0.2 mmol), 2a (1.2 equiv), PC-I (1 mol%), P-A (30 mol%), FeI 2 (15 mol%), K 2 HPO 4 (0.5 equiv), PhSiH 3 (1 mmol), MeCN (4 ml), blue LEDs, ambient temperature, 24-40 h. Full size image Subsequently, we studied the scope of the organonitro compounds (Fig. 3 ). A number of different nitroarenes can be successfully employed for selective formation of desired amides ( 3ss-3ax ). Both electron-donating and withdrawing groups on the phenyl rings barely influence the reaction efficiency, delivering the desired products in yields of up to 97%. Importantly, when the nitroarenes bearing nucleophilic functional groups, such free amino ( 3uu ), hydroxy ( 3al ), NH-free indole ( 3ao ), the amide bond formation between carboxylic acid and nitro groups is still predictable. These are cases which are challenging for classical amidation strategies with coupling reagents or transition metal-catalyzed aminocarbonylation [53] , [54] , [55] . There is also good functional group tolerance for nitroarenes. The aldehyde ( 3af ), ketone ( 3ae ), halogen ( 3tt , 3ac , 3ad , 3ah , 3ap ), heteroarene ( 3an , 3ao ) and Bpin ( 3ab ) are quite compatible. The use of nitroalkanes, such as nitromethane, nitroethane, nitropropane and nitrocyclopentane can successfully result in isolation of the desired amides (3aq-3ax ) in acceptable yields of 47–72%. Fig. 3: The scope of the organonitro compounds. Standard conditions: 1a (0.2 mmol), R-NO 2 2 (0.24 mmol), PC-I (1 mol%), P-A (30 mol%), FeI 2 (15 mol%), K 2 HPO 4 (0.5 equiv), PhSiH 3 (1 mmol), MeCN (4 ml), blue LEDs, ambient temperature, 24-36 h. a 2.0 equivalent nitromethane was used. Full size image Synthetic application To further demonstrate the synthetic robustness of Umpolung amidation, we used this amide bond formation strategy with complex molecules (Fig. 4a ). The excellent functional group tolerance and high selectivity of the reaction supports a predictable amide bond formation method. Complex carboxylic acids derived from AD-Acid ( 3ay ), ambrisentan ( 3az ), acolen ( 3ba ), actiprofen ( 3bc ), acemetacin ( 3bd ), etodolac ( 3be ), gluconorm ( 3bf ) and aminocyclo-propanecarboxylic acid ( 3bg ) are produced smoothly. Complex nitroarenes can also be successfully subjected to this Umpolung amidation reaction, affording for example, the desired product ( 3bh ) in 61% yield. 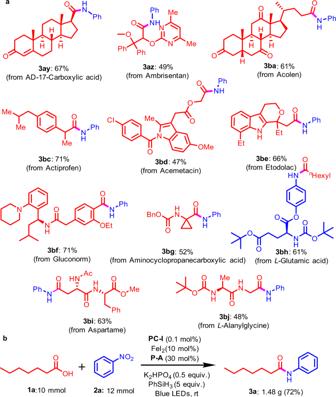Fig. 4: Synthetic application. aLate-stage Umpolung amidation of complex molecules. Standard conditions for late-stage modification: carboxylic acids1(0.2 mmol), nitroarenes2(0.24 mmol),PC-I(1 mol%),P-A(30 mol%), FeI2(15 mol%), K2HPO4(0.5 equiv), PhSiH3(1 mmol), MeCN (4 ml), blue LEDs, 24-60 h.bGram-scale test with 0.1 mol% photocatalyst. Standard conditions for gram-scale experiment:n-heptanoic acid1a(10 mmol), nitrobenzene2a(12 mmol),PC-I(0.1 mol%),P-A(30 mol%), FeI2(10 mol%), K2HPO4(0.5 equiv), PhSiH3(5 equiv), MeCN (100 ml), blue LEDs, 48 h. 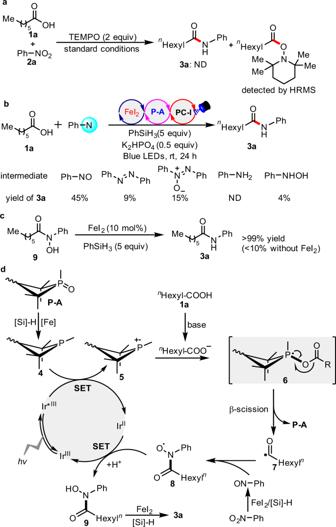Fig. 5: Mechanistic studies and proposed mechanism. aRadical inhibition experiment.bPotential N-based intermediate.cReduction of9to product3a.dProposed mechanism. Importantly, it was found that this protocol can be compatible for the late-stage modification of some peptides. Under the standard conditions, the carboxylic acid group in dipeptides of aspartame and L -alanylglycine can be employed for construction of amide bond in moderate isolated yields ( 3bi and 3bj ). The success of these complex molecules suggests the potential application of the Umpolung amidation method in the late-stage modification of complex molecules. Furthermore, with modified standard conditions using only 0.1 mol% photocatalyst, a scaled-up experiment of 10 mmol can be conducted smoothly to afford the desired product in 72% yield (Fig. 4b ). Fig. 4: Synthetic application. a Late-stage Umpolung amidation of complex molecules. Standard conditions for late-stage modification: carboxylic acids 1 (0.2 mmol), nitroarenes 2 (0.24 mmol), PC-I (1 mol%), P-A (30 mol%), FeI 2 (15 mol%), K 2 HPO 4 (0.5 equiv), PhSiH 3 (1 mmol), MeCN (4 ml), blue LEDs, 24-60 h. b Gram-scale test with 0.1 mol% photocatalyst. Standard conditions for gram-scale experiment: n -heptanoic acid 1a (10 mmol), nitrobenzene 2a (12 mmol), PC-I (0.1 mol%), P-A (30 mol%), FeI 2 (10 mol%), K 2 HPO 4 (0.5 equiv), PhSiH 3 (5 equiv), MeCN (100 ml), blue LEDs, 48 h. Full size image Mechanistic studies The following control experiments were performed to gain insight the mechanism of the reaction (Fig. 5 ). Under the standard conditions, upon addition of 2 equiv of TEMPO (2,2,6,6-tetramethylpiperidine-1-oxyl radical) into the reaction mixture, the reaction was completely inhibited and the corresponding acyl radical was trapped by TEMPO (Fig. 5a ), giving a product which was identified by high resolution mass spectroscopy (HRMS). In general, with the use of nitroarenes as electrophilic reagents, there are several kinds of potential N-based intermediates [27] , [50] , [52] , [56] , [57] . Among the potential intermediates that were screened, we found that the use of nitrosobenzene under experimental conditions could afford the desired product ( 3a ) in 45% yield, whereas the other electrophilic N-based intermediates such as 1,2-diphenyldiazene-1-oxide gave only a little product (Fig. 5b ). This suggests that nitrosobenzene potentially is the intermediate which reacts with the nucleophilic acyl radical. The use of aniline failed to generate the product ( 3a ) but N -phenylhydroxylamine gave 4% of the desired product (Fig. 5c ). We envisioned that the photoredox conditions with [*Ir(dF(CF 3 )ppy) 2 (dtbbpy)]PF 6 [ 1/2 E red (*Ir III /Ir II ) = + 1.21 V] [58] would slowly oxidize N -phenylhydroxylamine to the corresponding nitrosobenzene. In addition, under FeI 2 catalysis together with PhSiH 3 , the prepared intermediate ( 9 ), which can also be detected by HRMS in the reaction mixture, can directly be reduced to the final amide ( 3a ). In the light of previous work [32] , [33] , [34] , [35] , [36] , [37] , a plausible mechanism was proposed and is shown in Fig. 5d . After irradiation with blue LEDs, the excited photocatalyst [*Ir(dF(CF 3 )ppy) 2 (dtbbpy)]PF 6 [ 1/2 E red (*Ir III /Ir II ) = + 1.21 V] [58] causes a single electron oxidation of electron-rich R 3 P ( 4 ), which can be formed by reduction in situ from the precatalyst R 3 P = O ( P-A ) in the presence of PhSiH 3 and FeI 2 , generating the corresponding phosphine radical cation species ( 5 ). The Stern-Volmer quenching experiments demonstrated that the photoexcited [*Ir(dF(CF 3 )ppy) 2 (dtbbpy)]PF 6 could be quenched by R 3 P rather than R 3 P = O ( P-A ), n -heptanoic acid ( 1a ) or nitrobenzene ( 2a ). Subsequently, this species ( 5 ) can recombine with the carboxylate anion to furnish the radical intermediate ( 6 ). Owing to the high affinity of P- and O-atoms, intermediate ( 6 ) prefers to undergo β-scission to generate nucleophilic acyl radical ( 7 ) and complete the organophosphine catalytic cycle. Under the reductive reaction conditions with FeI 2 , the nitrobenzene ( 2a ) tends to form nitrosobenzene. Once the concentration of nitrosobenzene is relatively high, rapid nucleophilic acyl radical addition to nitrosobenzene occurs readily to give rise to N-centered radical intermediate ( 8 ). Donation of one electron to the Ir(II)-species would generate intermediate ( 9 ), completing the photoredox cycle. Finally, our control experiment showed that reduction of intermediate ( 9 ) with FeI 2 /PhSiH 3 to amide ( 3a ) at ambient temperature was almost quantitative. Less than 10% of amide ( 3a ) was obtained under the identical conditions without the addition of catalytic amount of FeI 2 . Fig. 5: Mechanistic studies and proposed mechanism. a Radical inhibition experiment. b Potential N-based intermediate. c Reduction of 9 to product 3a . d Proposed mechanism. Full size image We have developed an unprecedented synergistic catalysis system of iron/P(V-III)/photoredox catalysis for Umpolung amidation of carboxylic acids and nitroarenes or nitroalkanes. A wide range of commercially abundant and inexpensive carboxylic acids and nitroarenes are competent coupling partners in this direct amidation, affording a rich library of structurally diverse amides in yields of up to 97%. This amidation strategy surpasses the classical amide bond-forming method via carboxylic acid activation and subsequent amidation with nucleophilic amines, thus creating promising synthetic robustness especially when the substrates already have several sensitive functional groups or competing nucleophilic substituents. This protocol is readily scaled-up with 0.1 mol% photocatalyst for preparative systems. The excellent functional group compatibility and reaction selectivity render it useful in future peptide modification and drug discovery. General procedure for amidation To an 8 mL transparent vial equipped with a stirring bar, P-A (10.4 mg, 30 mol%), PC-I (2.2 mg, 1 mol%), FeI 2 (9.3 mg, 15 mol%), K 2 HPO 4 (17.4 mg, 0.1 mmol) were added successively. Then the vial was carried into glovebox which was equipped with nitrogen. Then MeCN (4.0 ml), PhSiH 3 (1 mmol), carboxylic acids 1 (0.2 mmol) and nitroarenes 2 (0.24 mmol) were added in sequence under N 2 atmosphere. The reaction mixture was stirred under the irradiation of 45 W blue LEDs (distance app. 10.0 cm from the bulb) at ambient temperature for 24–60 h. When the reaction finished, the mixture was quenched with water and extracted with ethyl acetate (3 × 10 mL). The organic layers were combined and concentrated under vacuo. The product was purified by flash column chromatography on silica gel (eluent: n- hexane: ethyl acetate).